Semiconducting single-walled carbon nanotubes sorting with a removable solubilizer based on dynamic supramolecular coordination chemistry Highly pure semiconducting single-walled carbon nanotubes (SWNTs) are essential for the next generation of electronic devices, such as field-effect transistors and photovoltaic applications; however, contamination by metallic SWNTs reduces the efficiency of their associated devices. Here we report a simple and efficient method for the separation of semiconducting- and metallic SWNTs based on supramolecular complex chemistry. We here describe the synthesis of metal-coordination polymers (CP-Ms) composed of a fluorene-bridged bis -phenanthroline ligand and metal ions. On the basis of a difference in the ‘solubility product’ of CP-M-solubilized semiconducting SWNTs and metallic SWNTs, we readily separated semiconducting SWNTs. Furthermore, the CP-M polymers on the SWNTs were simply removed by adding a protic acid and inducing depolymerization to the monomer components. We also describe molecular mechanics calculations to reveal the difference of binding and wrapping mode between CP-M/semiconducting SWNTs and CP-M/metallic SWNTs. This study opens a new stage for the use of such highly pure semiconducting SWNTs in many possible applications. Single-walled carbon nanotubes (SWNTs) possess a unique one-dimensional (1D) structure with remarkable electronic, mechanical, thermal and photophysical properties. Not only their structural characteristics, but also opto-electronic properties derived from their diameters and chiral indices, denoted as (n,m)SWNTs, are important for a deep understanding of their fundamental intrinsic properties [1] , [2] , [3] , [4] , [5] , [6] , [7] , [8] , [9] , [10] . Highly purified semiconducting SWNTs (sem-SWNTs) not containing metallic SWNTs (met-SWNTs) are specifically required for electronic devices, such as field-effect transistors [11] , [12] , [13] , [14] and photovoltaic applications [15] , [16] because the met-SWNTs decrease and reduce the efficiency of their associated devices [17] , [18] . Hence, the separation/purification of SWNTs according to their chirality is one of the most important issues in the science of carbon nanotubes. Such approaches can be simply classified into two ways containing the covalent- and non-covalent functionalization of the SWNT sidewalls [19] . In order to preserve the intrinsic SWNT properties, the latter method has an advantage over the former one. Recently, various methods for the separation of sem- and met-SWNTs including wrapping by SWNT solubilizers, such as DNAs [20] , [21] and π-conjugated or non-conjugated copolymers [11] , [22] , [23] , [24] , density gradient ultracentrifugation [25] , [26] and gel chromatography techniques [12] , [14] , [27] , [28] , [29] , [30] , [31] , [32] , [33] , [34] , [35] , [36] , [37] , [38] , [39] , have been reported. However, the reported techniques are rather complex and the efficiency is not very high. Polyfluorene-based copolymers (PFOs) [30] , [31] have been intensively studied because they dissolve/extract only sem-SWNTs in toluene by a simple sonication method. We have previously demonstrated a rational method for the selective extraction of a specific chirality of the sem-( n,m ) SWNTs using a series of systematically designed fluorene-based copolymers [32] , [33] , [34] . Moreover, we revealed that the PFO copolymers with a bulky optically active moiety could separate the right- and left-handed sem-SWNTs [35] . However, there are several serious problems when using PFOs; that is, difficulty in the removal of the wrapped PFOs from the SWNT/PFO composites [36] , [37] as well as their low extraction efficiency from the as-produced SWNTs [30] , [31] . The use of coordination bond formation is a facile and effective way to synthesize one-dimensional coordination polymers (CPs) with well-regulated geometries around metal ions by a simple bottom-up self-assembly method [38] , [39] . One of the most important features of such CPs is reversible bond formation (polymerization) and depolymerization to the monomer components by an outer stimulus, such as the addition of an acid, change in pH or temperature, photoirradiation, and so on [40] , [41] . Here we describe the separation of the sem- and met-SWNTs based on a supramolecular approach. As the goal, we design molecules (solubilizers) that efficiently recognize/solubilize sem-SWNTs based on the difference in the ‘solubility product’ between the sem- and met-SWNTs followed by detachment of the solubilizers from the SWNT surfaces to achieve simple and efficient separation of sem- and met-SWNTs from the pristine SWNTs, tunable selectivity by varying the components in the CPs, and simple removal of the solubilizers from the SWNT surfaces and possible reuse of them in the next sorting experiment. The chemical structures of these molecules are CPs composed of fluorene moieties and metal complexes, shown in Fig. 1 as PhenFO and CP-M , in which PhenFO , CP and M denote the phenanthroline (ligand for metal)-fluorene moiety, CP and metal ions, respectively. The fluorene backbone acts as the sem-SWNT recognition moiety and the phenanthroline-based metal complexes form polymers via coordination bonding. We report in this study the synthesis of PhenFO and CP-M (M=Co(II), Ni(II), Cu(II) and Zn(II) ions), efficient solubilization of SWNTs, separation of sem- and met-SWNTs from their mixture based on selective met-SWNT sedimentation and removal of CP-M to provide highly pure sem-SWNTs together with met-enriched SWNTs (see Fig. 1 ). Mayer and coworkers [42] and Chan-Park and coworkers [43] reported the use of degradable PFO-alternating copolymers, with a photocleavable or acid-sensitive moiety, to irreversibly cleave the wrapping polymers in order to remove them from the composites. Although they could obtain the sem-SWNTs as bundles, the purity of the sem-SWNTs was rather low and complete removal of the wrapping polymer was not discussed. Other groups have reported the solubilization of SWNTs based on the formation/deformation of supramolecules on the sidewall of SWNTs [44] , [45] ; however, their target was not selective sem- and met-SWNT separation. 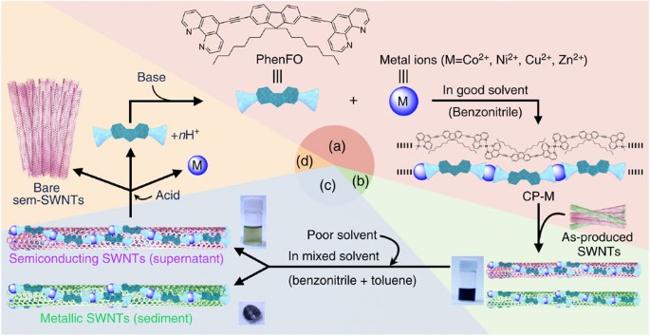Figure 1: A method for sem-SWNT sorting using removable solubilizers. The purification method starts from (a) the preparation ofCP-M(M=Co, Ni, Cu and Zn), (b) solubilization of as-produced SWNTs, (c) separation of sem- and met-SWNTs, and (d) removal and recovery of the adsorbents. Chemical structure ofPhenFOis shown in step a. Figure 1: A method for sem-SWNT sorting using removable solubilizers. The purification method starts from (a) the preparation of CP-M (M=Co, Ni, Cu and Zn), (b) solubilization of as-produced SWNTs, (c) separation of sem- and met-SWNTs, and (d) removal and recovery of the adsorbents. Chemical structure of PhenFO is shown in step a. Full size image Synthesis of CP-M The phenanthroline moiety is known to accept various metal ions [46] . We examined the coordination of PhenFO with the perchlorate salts of Co(II), Ni(II), Cu(II) and Zn(II) ions using the titration spectral change upon the addition of the metal ion into the solutions of PhenFO in benzonitrile. On the basis of the Job plots of each absorption maximum at 379, 387 and 410 nm as a function of the ratios of PhenFO and Cu(II) ion ( Supplementary Fig. 1 ), we found that a linear polymer was formed at metal:ligand=1:1 via coordination bonding [39] . Similar behaviour was observed when using Co(II), Ni(II) and Zn(II) in place of Cu(II) ( Supplementary Fig. 2 ). Solubilization of SWNTs by CP-M We first used benzonitrile as the solvent, since this is a good solvent for CP-M . In this solvent, CP-M was found to dissolve the SWNTs, but it dissolved both the sem- and met-SWNTs. It is known that PFOs exhibit selective sem-SWNT sorting only when aromatic solvents, such as toluene and xylene, are used [47] . However, the use of such solvents was difficult because of the poor solubility of the CP-M in such solvents. We thus tested mixed solvents of toluene/benzonitrile with the volume ratios of 1/3, 1/1 and 3/1; however, such mixed solvents did not dissolve CP-M . In order to obtain homogeneously dispersed SWNT solutions, we added a benzonitrile solution of PhenFO to equimolar metal ion solutions to prepare the CP-M in benzonitrile, to which the SWNTs were subsequently added and sonicated for 1 h, and then centrifuged at 10,000 g for 1 h, followed by collection of the upper 80% of each supernatant. As shown in Fig. 2a , absorbance (optical path length=1 mm) of the CP-M -solubilized SWNTs in the range of the first (S 11 ) and the second (S 22 ) semiconducting exciton bands reached 0.4 (M=Co), 0.3 (M=Fe), 0.2 (M=Cu) and 0.2 (M=Zn), which are ~20–40 times greater than that achieved when using conventional polyfluorenes, such as, poly(9,9-di-n-octylfluorenyl-2,7-diyl) in benzonitrile ( Supplementary Fig. 3 , optical length=1 cm). 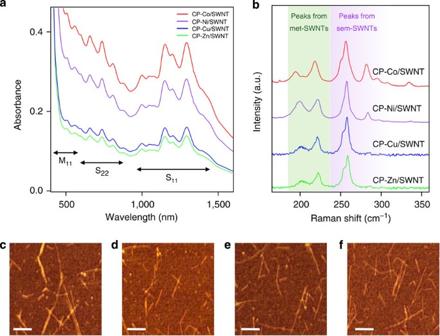Figure 2: Characterization of individualized SWNTs by the aid of CP-M in benzonitirile. (a) Vis-near infrared absorption spectra (optical cell length, 1 mm) and (b) Raman spectra for the RBM region of SWNTs (green-coloured area for met-SWNTs and purple-coloured area for sem-SWNTs with the excitation wavelength of 633 nm) of the solubilized SWNTs usingCP-M(M=cobalt(II) (red), nickel(II) (purple), copper(II) (blue), and zinc(II) (green) ions). (c–f). Atomic force microscopy images of the individually dispersed SWNTs wrapped with (c)CP-Co, (d)CP-Ni, (e)CP-Cuand (f)CP-Zn. Substrates used were mica. Scale bars, 200 nm. Figure 2: Characterization of individualized SWNTs by the aid of CP-M in benzonitirile. ( a ) Vis-near infrared absorption spectra (optical cell length, 1 mm) and ( b ) Raman spectra for the RBM region of SWNTs (green-coloured area for met-SWNTs and purple-coloured area for sem-SWNTs with the excitation wavelength of 633 nm) of the solubilized SWNTs using CP-M (M=cobalt(II) (red), nickel(II) (purple), copper(II) (blue), and zinc(II) (green) ions). ( c – f ). Atomic force microscopy images of the individually dispersed SWNTs wrapped with ( c ) CP-Co , ( d ) CP-Ni , ( e ) CP-Cu and ( f ) CP-Zn . Substrates used were mica. Scale bars, 200 nm. Full size image The absorption intensities of the solubilized SWNTs were found to increase in ascending order of atomic number of the used metal ions on the CP-M ( Fig. 2a ). According to coordination chemistry, cobalt(II) and nickel(II) ions are expected to form a square–planar structure on CP-M , while copper(II) and zinc(II) ions form a tetrahedral structure [48] . The difference in such coordination geometry may explain the difference in the amounts of the dissolved SWNTs. However, as shown in Fig. 2b , the Raman spectra of the solubilized SWNTs were shown to contain both sem- and met-SWNTs and therefore the separation was unsuccessful at this stage (for the Raman spectra in the range of 500–2,000 cm −1 excited at 633 nm and the spectra obtained with 532-nm- and 785-nm excitation, see Supplementary Figs 4–6 ). To obtain the structure of the solubilized SWNTs, we carried out atomic force microscopy measurements of SWNT/ CP-M composites (for M=Co, Ni, Cu and Zn; Fig. 2c–f ) and the results for their height distribution are shown in Supplementary Fig. 7 , in which we observe SWNTs with heights (average for each 100 points) of 1.2±0.1 nm for M=Co, Ni, Cu and Zn, suggesting individual dissolution of the SWNTs in all samples. Such height values agree with those of the optimized structures that we discuss in the molecular mechanics calculation section. Separation of sem-SWNTs and met-SWNTs We now describe how to separate the sem- and met-SWNTs from their mixtures. We discovered that the ‘solubility product’ [49] was different for the CP-M -wrapped sem-SWNTs and met-SWNTs such that the addition of toluene (50 vol%) to the benzonitrile solutions of the SWNT- CP-M (M=Co, Ni, Cu or Zn) caused precipitates. Under ambient conditions, the concentrations of the SWNTs in the supernatant solutions reached equilibrium in 12 h. Interestingly, we found that only the sem-SWNTs remained in the supernatants and the met-SWNTs were enriched in the sediments. We call this technique a ‘solubility product’ method for the separation of sem- or met-SWNTs. The four different supernatants including the SWNT- CP-M (M=Co, Ni, Cu or Zn) were filtered to remove the excess CP-M , and the obtained residues were used for Raman spectral measurements. We also measured the vis-near infrared (NIR) spectra of the residues that were completely redissolved in benzonitrile. The results are shown in Fig. 3 (for the Raman spectra in the range of 500–2,000 cm −1 excited using 633-nm laser and the Raman spectra measured using 532-nm- and 785-nm laser excitation, see Supplementary Figs 8–10 , respectively). 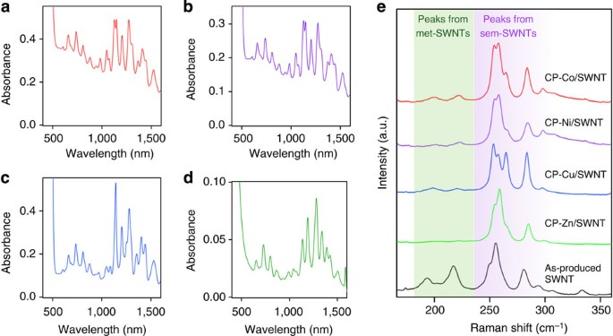Figure 3: Vis-NIR absorption and Raman spectra of the supernatant solutions obtained after the ‘solubility product’ method. (a–d) Vis-NIR absorption spectra of sorted sem-SWNTs using CP-Co (a), CP-Ni (b), CP-Cu (c) and CP-Zn (d) in the supernatant obtained after the addition of toluene (50 vol%) into the SWNT solutions in benzonitrile (optical cell length: 2 mm). (e) Raman spectra (excitation wavelength: 633 nm) of the solids obtained by filtration of the supernatant solutions. Raman spectrum of the pristine HiPco-SWNTs is also shown for comparison (black line). Figure 3: Vis-NIR absorption and Raman spectra of the supernatant solutions obtained after the ‘solubility product’ method. ( a – d ) Vis-NIR absorption spectra of sorted sem-SWNTs using CP-Co ( a ), CP-Ni ( b ), CP-Cu ( c ) and CP-Zn ( d ) in the supernatant obtained after the addition of toluene (50 vol%) into the SWNT solutions in benzonitrile (optical cell length: 2 mm). ( e ) Raman spectra (excitation wavelength: 633 nm) of the solids obtained by filtration of the supernatant solutions. Raman spectrum of the pristine HiPco-SWNTs is also shown for comparison (black line). Full size image Notably, by comparison with the absorption spectra shown in Fig. 2a , we recognized the disappearance of the met-SWNT bands ~450–600 nm ( Fig. 3a–d ). The UV–vis-near-IR absorption spectrum of the purified sem-SWNTs dispersed using an sodium dodecylsulfate (SDS) aqueous solution is shown in Fig. 4f , in which we recognize that the spectrum is not suitable to determine the ratio of met- and sem-SWNTs. The Raman spectra provided proof of the separation of the met- and sem-SWNTs [50] , [51] , [52] . For the HiPco-produced SWNTs, based on the Kataura plot [53] , [54] , we can estimate the ratio of the sem- or met-SWNTs using the RBM region in the Raman spectra measured by excitation at 633 nm, which is a widely used method [31] , [36] , [43] , [55] . Compared with the spectrum of the as-produced SWNTs (black line in Fig. 3e ), the metallic band around 180–240 cm −1 greatly decreased in the spectra of the CP-M -SWNTs obtained after the ‘solubility product’ procedure ( Fig. 3e ), indicating that the purity of the sem-SWNTs was very high. 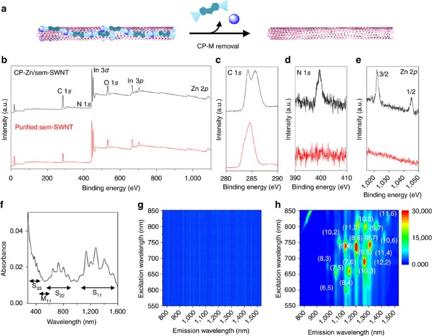Figure 4: Validation of CP-M removal from SWNT surfaces. (a) Schematic illustration of the removal ofCP-Mfrom the sem-SWNT surfaces via depolymerization of theCP-M. (b–e) XPS of the SWNTs before (black line) and after (red line) the depolymerization procedure of theCP-Zn/sem-SWNT composites. Narrow scans for (c) carbon (C 1s), (d) nitrogen (N 1s) and (e) zinc (Zn 2p) is also shown. Carbon peak in the originalCP-Zn/sem-SWNT composites consists of two peaks of 284.3 eV for SWNT and 285.5 eV forCP-Zn, while after the removal process only 284.5 eV peak is observed. Disappearance of the peaks of nitrogen and zinc after the depolymerization procedure indicates a successful removal ofCP-M. The number of scans is 5 for survey scan, 3 for carbon, 10 for nitrogen and 20 for zinc. Samples were fixed on indium plate. (f) UV–vis-NIR absorption of purified sem-SWNTs dispersed using SDS in D2O. SWNT absorption region ranges fromEs11Es22Es33for sem-SWNTs andEmfor met-SWNTs are denoted. (g,h) two-dimensional photoluminescence mappings of the SDS-solubilized SWNTs before (g) and after (h) the removal ofCP-Zn. Figure 4: Validation of CP-M removal from SWNT surfaces. ( a ) Schematic illustration of the removal of CP-M from the sem-SWNT surfaces via depolymerization of the CP-M . ( b – e ) XPS of the SWNTs before (black line) and after (red line) the depolymerization procedure of the CP-Zn /sem-SWNT composites. Narrow scans for ( c ) carbon (C 1 s ), ( d ) nitrogen (N 1 s ) and ( e ) zinc (Zn 2 p ) is also shown. Carbon peak in the original CP-Zn /sem-SWNT composites consists of two peaks of 284.3 eV for SWNT and 285.5 eV for CP-Zn , while after the removal process only 284.5 eV peak is observed. Disappearance of the peaks of nitrogen and zinc after the depolymerization procedure indicates a successful removal of CP-M . The number of scans is 5 for survey scan, 3 for carbon, 10 for nitrogen and 20 for zinc. Samples were fixed on indium plate. ( f ) UV–vis-NIR absorption of purified sem-SWNTs dispersed using SDS in D 2 O. SWNT absorption region ranges from E s [11] E s [22] E s [33] for sem-SWNTs and E m for met-SWNTs are denoted. ( g,h ) two-dimensional photoluminescence mappings of the SDS-solubilized SWNTs before ( g ) and after ( h ) the removal of CP-Zn . Full size image When using the CP-M (M=Co and Ni), the extracted sem-purity was lower than those using CP-M (M=Zn and Cu). As shown in Fig. 2a , the amounts of SWNTs dissolved by CP-M (M=Co and Ni) were much greater than those using the CP-M (M=Cu and Zn). The degree of the sem-SWNT selectivity and the amounts of the extracted SWNTs might be related [47] . Such behaviour is understandable, since it is expected that greater amounts of solubilized SWNTs may undergo a loss of the high sem-/met-SWNT sorting selectivity. The sediments generated by the ‘solubility product’ procedure were also analysed. They were fully dissolved in benzonitrile by sonication for 30 min. On the basis of their absorption and Raman spectra ( Supplementary Figs 11–14 , respectively), the met-SWNTs were greatly enriched in the solutions compared with the as-produced SWNTs, namely, the determined met-SWNT/sem-SWNT ratios were 3/1, 2/1, 1/1 and 1/1 for CP-Co , CP-Ni , CP-Cu and CP-Zn , respectively, which were greater than that of the as-produced SWNT (met-SWNTs/sem-SWNTs=3/7). The observed metal dependency on the met-SWNT enrichment is related to the initial amounts of the solubilized SWNTs. Removal of the CP-M As mentioned above, removal of the SWNT adsorbents (solubilizers) is essential for the efficient use of sem- and met-SWNTs in many applications. We now focus on how to produce pure sem-SWNTs by the removal of CP-M from the CP-M /sem-SWNT composites. When using conventional PFOs and their copolymers, their removal from the SWNT composites is quite difficult because of the strong interactions between the PFOs and SWNTs. The removal of adsorbents in our samples, on the other hand, was quite simple because the adsorbents are not covalent polymers but CPs, which are readily depolymerized to the corresponding monomer units by the addition of an acid [40] . Eventually, the addition of a large excess trifluoroacetic acid to the supernatants generated precipitates, which were filtered, rinsed with benzonitrile and then with methanol, followed by air-drying. The obtained solids were analysed using X-ray photoelectron spectroscopy (XPS) and the result is shown in Fig. 4b–e , in which no peak of the metal ions and nitrogen appeared, indicating complete removal of the CP-Zn . The XPS of before and after the polymer removal process on CP-M (M=Co, Ni and Cu)/SWNT are shown in Supplementary Figs 15–17 . All these results clearly indicate that the metal ions and PhenFO of the CP-M (M=Co, Ni, Cu and Zn) were completely removed from their complexes with the sem-SWNTs. The four different solids obtained after the removal of CP-M (M=Co, Ni, Cu and Zn) were each dispersed in 1 wt% SDS aqueous micelle solutions in order to confirm the removal of the CP-M together with the determination of the (n,m) chiralities based on the analysis of their two-dimensional photoluminescence mappings. As shown in Fig. 4g , CP-M completely quenched the PL of the SWNTs before acid treatment because of the well-known heavy atom effect [56] . Following acid treatment, however, we observed evident PL signals for the SDS-redispersed samples, which is direct evidence that the CP-Zn was removed from the CP-Zn /SWNT composite ( Fig. 4h ). The same behaviour was observed when CP-M (M=Co, Ni and Cu) was used in place of CP-Zn ( Supplementary Fig. 18 ). The removal of the CP components was also confirmed using UV–vis-NIR absorption ( Fig. 4f ) and Raman ( Supplementary Figs 19–21 ) spectroscopies. It was revealed that no absorption of PhenFO (absorption max, 375 nm) and CP-M (absorption range, 360–400 nm) was recognized, which is direct proof of the removal. We can now readily determine the (n,m) SWNT chiralities from the PL-mapping. As shown in Fig. 4h , sem-SWNTs with (n,m)=(6,5), (7,5), (7,6), (8,3), (8,4), (8,6), (8,7), (9,4), (9,5), (9,7), (10,2), (10,3), (10,5), (10,6), (11,3), (11,4), (11,6) and (12,2) were found to exist in the solution. In order to evaluate the extraction efficiency for each (n,m) chirality of the tubes, we calculated the relative contents of each SWNT based on the calibrated PL intensity using the method reported by Oyama et al . [57] The calibrated contents of the SWNT species deduced from the PL mapping are shown in Supplementary Table 1 , in which SWNTs with (n,m)=(7,6), (8,6), (9,4) and (10,2) were enriched for the sample using CP-Zn . We also calculated the calibrated contents for the samples using CP-M (M=Co, Ni and Cu; Supplementary Tables 2–4 ). The removed PhenFO molecules in the acid treatment were quantitatively deprotonated under basic conditions, indicating that reuse of the recovered CP-M for a further SWNT solubilization experiment is possible, which is another significant advantage of our method. Finally, we discuss the extraction/separation efficiency of our ‘solubility product’ method. On the basis of the decrease in the absorbance intensity between the sample solutions before and after the ‘solubility product’ method, the sem-SWNT sorting efficiencies were 66, 57, 91 and 32% for CP-Co , CP-Ni, CP-Cu and CP-Zn , respectively. By repeating the ‘solubility product’ method for the precipitates, such efficiency is expected to be enhanced. We emphasize that the present method is simple and efficient for the separation of the sem- and met-SWNTs. It is also expected that by changing the metal ions, counter anions, solvents and ligands, a more efficient selective collection of the sem-SWNTs with a specific chirality might be possible. Molecular mechanics simulations As described above, CP-Zn sorted the sem-SWNTs with a very high efficiency (especially, sem-(8,6) SWNTs, see Supplementary Table 1 ), while CP-Co did not. In an effort to understand these recognition differences, a computer simulation technique was used to model the sem-(8,6)- and met-(7,7) SWNTs as the typical sem- and met-SWNTs, respectively, since their diameters are close (0.952 and 0.949 nm for (8,6)- and (7,7) SWNTs, respectively). We carried out an all-atomic molecular mechanical calculation using the OPLS2005 force field [58] . The used initial structure of the CP-M strip was a 6-mer (oligomer), which was found in the electrospray ionization-time of flight (ESI-TOF)-mass spectrum ( Supplementary Fig. 22 ). The length of each SWNT used in this calculation was 30 nm, which is efficient for the contact of the CP-Ms with the centre 1/3 of the SWNT. Considering the surface areas of the SWNTs, four different CP-M strips were placed to cover the SWNTs and were used as the initial structures. This model was equilibrated in toluene by simulation using a low-mode sampling and the structures were minimized using the OPLS2005 force field. We calculated the optimized structures for the combination of CP-Zn with sem-(8,6) SWNT ( Fig. 5a ), or met-(7,7) SWNT ( Fig. 5b ), as well as those of CP-Co with sem-(8,6) SWNT ( Fig. 5c ) or met-(7,7) SWNT ( Fig. 5d ). 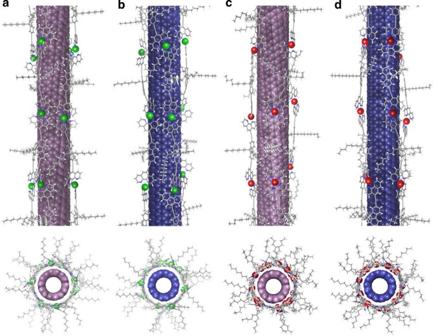Figure 5: Optimized structures of the simulated CP-M-wrapped SWNTs. (a–d) Top views (top row) and side views (bottom row) ofCP-Zn/sem-(8,6)-SWNT (a),CP-Zn/met-(7,7)-SWNT (b),CP-Co/sem-(8,6)-SWNT (c) andCP-Co/met-(7,7)-SWNT(d). Metal ions are represented as spheres highlighted in green for Zn(II) and red for Co(II), respectively. To predict the binding strengths between the CP-M and the (8,6)- and (7,7) SWNTs, the binding energies ( E stabilizing ) of each SWNT with the CP-M complex were calculated as: Figure 5: Optimized structures of the simulated CP-M-wrapped SWNTs. ( a – d ) Top views (top row) and side views (bottom row) of CP-Zn /sem-(8,6)-SWNT ( a ), CP-Zn /met-(7,7)-SWNT ( b ), CP-Co /sem-(8,6)-SWNT ( c ) and CP-Co /met-(7,7)-SWNT( d ). Metal ions are represented as spheres highlighted in green for Zn(II) and red for Co(II), respectively. Full size image where E complex , E SWNT and E CP-M are the energies of the SWNT/ CP-M complexes, SWNT and CP-M , respectively [32] , [59] , [60] . The results are summarized in Table 1 for the calculated potential and stabilizing energy of the CP-Co and CP-Zn systems, respectively. Table 1 Calculated potential and stabilizing energies between the (n,m) SWNTs with the CP-M (M=Zn or Co) in solvents. Full size table In the simulations using toluene as the solvent, the stabilizing energy for the interaction between the CP-Zn and the sem-(8,6)SWNT was −5,404.7±9.9 kcal mol −1 , which is much higher than that between the CP-Zn and met-(7,7)SWNT (−4,331.9±3.8 kcal mol −1 ) and the stabilizing energies between the CP-Co with the (8,6)- and (7,7)SWNTs were comparable (−5,563.4±4.2 and 4567.4±19.8 kcal mol −1 , respectively). In the optimized simulated structure of CP-Zn /SWNT, the fluorene moieties semihelically aligned on both the sem-(8,6) and met-(7,7) SWNTs when the complexes take a tetrahedral configuration ( Fig. 5a,b , respectively). On the other hand, the square–planar complex of CP-Co preferred to take a straight configuration on the met-SWNT ( Fig. 5c,d ). This different recognition behaviour together with the obtained binding energies indicates that CP-Zn with a tetrahedral coordination structure favours sem-(8,6) SWNT rather than met-(7,7) SWNT in toluene, which is consistent with the experimental results. When using benzonitrile in place of toluene, the stabilizing energies of the met- and sem-SWNT complexes were not very different ( Table 1 and Supplementary Fig. 23 ). Furthermore, simulations using different initial configurations are also carried out using CP-Zn , in which all the alkyl chains wrap the SWNT sidewalls with no conjugated moieties that contact the SWNT ( Supplementary Fig. 24 and Supplementary Table 5 ). The result showed a lower stabilizing energy and no clear stabilizing energy difference between the sem-SWNT and met-SWNTs in both toluene and benzonitrile. By taking this conformation, the fluorene backbone can be more flexible to fit the curvature of the SWNT surface, which agreed with the report for the PFO simulations [47] . All these results suggested that the interactions of the fluorene backbone together with conjugated metal complex moiety to the SWNT side walls is important for the selective separation of sem- and met-SWNTs. In conclusion, a novel strategy for the efficient extraction of highly pure sem-SWNTs based on supramolecular coordination chemistry is presented. The most interesting features are summarized as follows: (i) we designed and synthesized coordination polymers CP-M (M=Co, Ni, Cu and Zn) that exhibited an excellent SWNT-solubilizing ability in benzonitrile, (ii) based on our ‘solubility product’ procedure, we isolated only the sem-SWNTs, (iii) we have succeeded in the complete removal of the wrapping CP-M by a simple acid treatment and (iv) the selectivity of the met- and sem-SWNTs was explained by molecular mechanics simulations. Such an efficient and easy extraction of the sem-SWNTs is a great advance in the chirality separation science of SWNTs and opens a new field for use of such materials in many applications. Materials All chemicals and solvents used in the syntheses were of reagent grade and used without further purification. 5-Bromo2,7-phenanthroline and 2,7-bisethynyl-9,9-dioctylfluorene were synthesized according to the literature [61] , [62] . Synthesis of 2,7-bis((1,10-phenanthrolin-5-yl)ethynyl)-9,9-dioctyl-9 H-fluorene ( PhenFO ) PhenFO was synthesized via the Sonogashira coupling ( Supplementary Fig. 25a ): 5-bromo2,7-phenanthroline (170 mg, 0.656 mmol), 2,7-bisethynyl-9,9-dioctylfluorene (141 mg, 0.322 mmol), tetrakis(triphenylphosphine)palladium (70 mg, 0.061 mmol), copper(I) iodide (19 mg, 0.010 mmol) and triethylamine (50 ml) were placed in a 100-ml-two-necked flask and stirred at 70 °C for 6 h under flowing nitrogen, and then cooled to room temperature and filtered. The filtrate was concentrated and purified using silica gel column chromatography eluted by dichloromethane. The first fraction was collected and recrystallized from hexane to provide PhenFO as yellow needle-like crystals. Yield: 86%. 1 H NMR (300 MHz, CDCl 3 ): δ 9.28 (d, J =4.3, 2H), 9.22 (d, J =4.3 2H), 8.92 (d, J =8.3 2H), 8.26 (d, J =8.2 2H), 8.17 (s, 2H), 7.80 (m, 4H), 7.70 (m, 4H), 7.66 (s, 2H), 2.09 (m, 4H), 1.26−1.06 (m, 20H), 0.80−0.66 (m, 10H). 13 C NMR (75 MHz, CDCl 3 ): δ 151.405, 150.930, 150.712, 146.178, 146.045, 141.200, 135.760, 134.812, 131.120, 130.658, 128.305, 128.144, 126.094, 123.513, 123.383, 121.547, 120.325, 120.106, 96.373, 86.401, 55.488, 31.778, 30.894, 29.987, 29.242, 29.205, 23.769, 22.579, 14.040. High-resolution mass spectroscopy (ESI, m/z ): [M+H + ] calcd. for C 57 H 55 N 4 , 795.0870; found, 795.0872 ( Supplementary Figs 25 and 26 ). General method for the preparation of CP-M A 3.0-ml portion of PhenFO (0.1 mM in benzonitrile) was added to an equimolar solution of the perchlorate salt of Co(II), Ni(II), Cu(II) or Zn(II) ion to immediately produce CP-M . A concentration-dependent titration of each metal ion in the PhenFO solution revealed that the PhenFO and each metal ion formed complexes with the molar ratios=1:1, indicating the formation of linear coordination polymers ( Supplementary Fig. 1 ). The molecular masses of the CP-M were measured by an ESI-TOF-Mass spectrometer (Bruker Co., Ltd., micrOTOF-QIII) and oligomers of up to 10-mer ([ PhenFO 10 M 9 (ClO 4 ) 9 ] 9+ ) were found in the benzonitrile solution ( Supplementary Fig. 22 ). General method for the solubilization of SWNTs The SWNTs (HiPco) were purchased from Unydim Co., Ltd. (Lot No. P0261) and used as received. A typical procedure for the SWNT dissolution using CP-M (M=Co, Ni, Cu or Zn) is as follows: crude SWNTs (1 mg) were dispersed in a 0.1-mM (for the PhenFO ) benzonitrile solution of CP-M (3 ml) using a bath-type sonicator (Emerson Japan Ltd., Bransonic) for 1 h, followed by centrifugation at 10,000 g for 1 h, and then the upper 80% of the supernatant was collected. The vis-NIR absorption spectra were measured using a spectrophotometer (JASCO Co., Ltd., type V-670). The PL spectra were measured by a spectrofluorometer (Horiba-Jobin Yvon, SPEX Fluorolog-3-NIR) equipped with a liquid-nitrogen-cooled InGaAs near-IR detector. The excitation and emission wavelengths were in the range of 500–900 and 900–1,300 nm, respectively. The Raman spectra at 532, 633 and 785 nm were recorded by a Raman spectrometer (Nanophoton Co., Ltd., Raman Touch). Atomic force microscopy images were taken using a scanning probe microscope (Agilent Technologies, type 5500). Mica was used as the substrate. XPS spectra were measured using an AXIS-ULTRA DLD (Shimadzu). Selective separation of sem- and met-SWNTs The obtained supernatants (2 ml each) were added to toluene (2 ml) followed by gentle swirling (caution: gentle swirling is important because vigorous stirring caused precipitation of all the SWNTs in the supernatant), and then kept overnight at room temperature. The obtained solution was centrifuged at 10,000 g for 1 h, and then the upper 80% of the supernatant was collected. After removing the lower 20% of the supernatant, the sediments were collected and then redispersed in benzonitrile to obtain a homogenized solution. Removal of CP-M from the solubilized SWNTs The obtained top-80% of the supernatant and the redispersed solutions of the sediments were filtered using PTFE filters (ADVANTEC, 0.1-μm pore size). Each collected solid was dispersed in 3 ml of benzonitrile to which a 0.5-ml proportion of trifluoroacetic acid (15 wt%, 4.4 mmol) was added to immediately generate a black suspension, which was filtered through a PTFE filter (ADVANTEC, 0.1-μm pore size) and washed with 10 ml of benzonitrile followed by washing with methanol until the absorption of CP-M disappeared in the UV–vis absorption spectrum of filtered liquid. Each obtained SWNT solid was redispersed in 3 ml of a 1 wt% SDS aqueous solution to measure their vis-NIR absorption, Raman, XPS and PL spectra. Molecular mechanics calculation The molecular mechanics simulations were carried out using MacroModel (Schrodinger, version 9.4) with the OPLS2005 force field. The dielectric constant of toluene (2.3) and benzonitrile (25.2) were used in the calculation. The charge of the complexes was assigned by the software and the counter anions were not placed. The initial structures were first fluctuated using molecular dynamics simulation in 300 K (MacroModel), and then three states were randomly chosen as the input structures for the molecular mechanics simulations. Minimization of the calculation was carried out using the Polak-Ribiere conjugate gradient with a convergence threshold on the gradient of 0.05 kJ mol −1 . Default values were used for all the other parameters. How to cite this article: Toshimitsu F. and Nakashima N. Semiconducting single-walled carbon nanotubes sorting with a removable solubilizer based on dynamic supramolecular coordination chemistry. Nat. Commun. 5:5041 doi: 10.1038/ncomms6041 (2014).